Reconstructing targetable pathways in lung cancer by integrating diverse omics data Global ‘multi-omics’ profiling of cancer cells harbours the potential for characterizing the signalling networks associated with specific oncogenes. Here we profile the transcriptome, proteome and phosphoproteome in a panel of non-small cell lung cancer (NSCLC) cell lines in order to reconstruct targetable networks associated with KRAS dependency. We develop a two-step bioinformatics strategy addressing the challenge of integrating these disparate data sets. We first define an ‘abundance-score’ combining transcript, protein and phospho-protein abundances to nominate differentially abundant proteins and then use the Prize Collecting Steiner Tree algorithm to identify functional sub-networks. We identify three modules centred on KRAS and MET, LCK and PAK1 and β-Catenin. We validate activation of these proteins in KRAS-dependent (KRAS-Dep) cells and perform functional studies defining LCK as a critical gene for cell proliferation in KRAS-Dep but not KRAS-independent NSCLCs. These results suggest that LCK is a potential druggable target protein in KRAS-Dep lung cancers. Activating mutations in the Ras oncogenes characterize 20–40% of all non-small cell lung cancer (NSCLC) [1] , [2] , [3] , the leading cause of cancer mortality in the United States [4] , which establishes Ras genes as the most commonly mutated oncogenes in this malignancy. KRAS, NRAS and HRAS, the main members of this family of GTPase proteins, are activated by somatic mutations in 20–30%, 1–5% and 1% of the NSCLC cases, respectively [1] . Mutated Ras has been implicated in activating numerous pathways that control cell proliferation and survival; however, development of drug therapies aimed at disrupting Ras activity has proved challenging [1] . Consequently, recent efforts have focused on identifying indirect mechanisms to disrupt Ras signalling by targeting either upstream activators or downstream effectors [5] , [6] , [7] , [8] , [9] . To this end, microarray gene expression profiling has been extensively used to define expression signatures characterizing Ras mutations in cell lines and tumours [10] , [11] , [12] , but gene signatures vary considerably across these studies. Complicating these initial studies, recent work has shown that NSCLCs with activating KRAS mutations can be stratified into KRAS-dependent (KRAS-Dep) or KRAS-independent (KRAS-Ind) groups according to their requirement for mutant KRAS signalling to sustain growth and proliferation [8] , [9] , [13] , [14] . Therefore, after shRNA knock down of KRAS, KRAS-Ind cells would grow at rates resembling cells treated with control shRNAs, whereas KRAS-Dep grow at slower rates. Here gene expression profiles of NSCLC cell lines found that KRAS dependency correlated with a differentiated phenotype, whereas KRAS independency was associated with the epithelial–mesenchymal transformation phenotype [13] , [14] . Moreover, recent work associated KRAS dependency with activation of the Wnt signalling pathway in colorectal cancers [14] . Taken together, these results suggest that specific pathways are activated in KRAS-Dep cell lines but not in KRAS-Ind cells, and that those pathways have a role in the varying disease phenotypes found in these cancers. While such expression profiling studies are useful for the analysis of KRAS signalling, it is well established that KRAS frequently exerts oncogenic functions through changes in protein abundance or post-translational modifications of proteins, specifically kinases that in turn induce a signalling cascade of downstream effectors [15] , [16] , [17] , [18] . Consequently, global transcriptome, proteome and phosphophospho-proteome profiling methods should be applied in order to identify causative pathways in KRAS-Dep and KRAS-Ind NSCLC cells in an unbiased fashion. However, to date no study has comprehensively integrated these diverse sets of data [5] , [10] , [11] , [15] , [17] , [18] , [19] , leading to potential biases and inadequacies in our understanding of the mechanistic basis for KRAS function in NSCLC. One reason why such studies are lacking is because integration of such diverse data sets is a major challenge with existing integrative methods. Yet when employed, integrative methods have been successful in building more comprehensive models of molecular signalling networks in cancer [20] , [21] . In this study, we generate a matched data set of KRAS-mutated NSCLC cell lines with global and unbiased transcriptome, proteome and phosphoproteome profiles. We develop a bioinformatics approach to integrate these disparate omics data sets and nominate biologically informative signalling modules using network analysis. We find that KRAS-Dep cell lines harbour an active and targetable sub-network composed of lymphocyte-specific tyrosine kinase ( LCK ), cMET , KRAS and the p21 serine/threonine activated kinase ( PAK1 ). We characterize a KRAS–LCK–PAK1 pathway and show that KRAS-Dep but not KRAS-Ind cell lines require LCK for proliferation. This KRAS–LCK–PAK1 network further coordinates anti-apoptotic pathways both through inhibition of pro-apoptotic proteins such as BAD and/or activation of anti-apoptotic proteins in KRAS-Dep cell lines. In summary, this study identifies active networks associated with the KRAS-Dep phenotype in NSCLC and nominates a novel KRAS–LCK–PAK1 pathway in KRAS-Dep cells that may serve as a druggable pathway for treating KRAS-Dep lung cancers. Omics integration improves the nomination of actionable proteins To study KRAS function in lung cancer, we generated matched global transcriptome, proteome and phosphoproteome data sets for a panel of KRAS-Dep and KRAS-Ind NSCLC cell lines, as well as a bioinformatics methodology to integrate all those data types ( Fig. 1a ). Transcript, protein and phospho-protein abundance were measured by microarrays and label-free LS-MS/MS respectively (Methods). We identified 3,213 proteins in the unmodified state and 1,044 proteins in the phosphorylated state, with at least one spectrum count in two independent cell lines. The number of unique peptides and phospho-peptides for each cell line are shown in the Supplementary Fig. S1A,B , and the full proteome and phosphoproteome data sets for all cell lines are given in Supplementary Data 1 and 2 and Supplementary Data 3 and 4 , respectively. 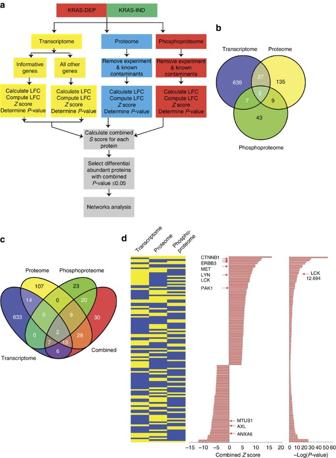Figure 1: Integrative analysis of omics data reveals targetable kinases in NSCLC KRAS-Dep cell lines. (a) A panel of KRAS-Dep and KRAS-Ind cell lines was analysed by transcriptomics, proteomics and phospho-proteomics techniques. Transcripts were split in two different categories: ‘informative’ genes and ‘all other’ genes. Proteome and phopho-proteome data sets were normalized with respect to the total number spectral counts in each library, and common contaminants and ‘Deja vu’ proteins were filtered out before quantification of differential abundance. All data sets were log-transformed and the LFC was taken with respect to the comparison KRAS-Dep versus KRAS-Ind cell lines. The LFC wasz-score-normalized and aP-value was calculated using the standard normal distribution. The combinedSscore was used to integrate all three data sets (methods) and select differentially expressed proteins. Network and enrichment analysis were performed using SPIA and the PCST. (b)Naive integration of data sets. Only~5.2% of the proteins are shared among two of the data sets (adjustedP-value0.05 was used as a threshold to select differentially expressed proteins). A major drawback of this method is the absence of an objective criterion to include proteins differentially expressed in only one data set. (c)A meta-integration of the independent signatures using the combinedSscore (S). TheSscore integration improves by fivefold the percentage of shared proteins among data sets (~26%) and defines an objective rule for including proteins differentially expressed in one, two or all data sets. (d)Integrative analysis of transcriptome, proteome and phospho-proteome nominates receptor tyrosine kinasesMETandERBB3, Src family membersLCKandLYN,PAK1, andCTNNB1,CTNNA1andCDH1among others as differentially ‘activated’ proteins in KRAS-Dep cell lines. Left: presence/absence heatmap. Proteins that are differentially abundant in a particular data set are represented in yellow and unaffected proteins are represented in blue. Middle: combinedSscore (S) for all differentially abundant proteins in KRAS-Dep versus KRAS-Ind cell lines. Right: combined statistical significance for each differentially abundant protein. −log of the Hochberg-adjustedP-value, −log(0.05)=1.30. Figure 1: Integrative analysis of omics data reveals targetable kinases in NSCLC KRAS-Dep cell lines. ( a ) A panel of KRAS-Dep and KRAS-Ind cell lines was analysed by transcriptomics, proteomics and phospho-proteomics techniques. Transcripts were split in two different categories: ‘informative’ genes and ‘all other’ genes. Proteome and phopho-proteome data sets were normalized with respect to the total number spectral counts in each library, and common contaminants and ‘Deja vu’ proteins were filtered out before quantification of differential abundance. All data sets were log-transformed and the LFC was taken with respect to the comparison KRAS-Dep versus KRAS-Ind cell lines. The LFC was z -score-normalized and a P -value was calculated using the standard normal distribution. The combined S score was used to integrate all three data sets (methods) and select differentially expressed proteins. Network and enrichment analysis were performed using SPIA and the PCST. ( b )Naive integration of data sets. Only~5.2% of the proteins are shared among two of the data sets (adjusted P -value 0.05 was used as a threshold to select differentially expressed proteins). A major drawback of this method is the absence of an objective criterion to include proteins differentially expressed in only one data set. ( c )A meta-integration of the independent signatures using the combined S score ( S ). The S score integration improves by fivefold the percentage of shared proteins among data sets (~26%) and defines an objective rule for including proteins differentially expressed in one, two or all data sets. ( d )Integrative analysis of transcriptome, proteome and phospho-proteome nominates receptor tyrosine kinases MET and ERBB3 , Src family members LCK and LYN , PAK1 , and CTNNB1 , CTNNA1 and CDH1 among others as differentially ‘activated’ proteins in KRAS-Dep cell lines. Left: presence/absence heatmap. Proteins that are differentially abundant in a particular data set are represented in yellow and unaffected proteins are represented in blue. Middle: combined S score ( S ) for all differentially abundant proteins in KRAS-Dep versus KRAS-Ind cell lines. Right: combined statistical significance for each differentially abundant protein. −log of the Hochberg-adjusted P -value, −log(0.05)=1.30. Full size image Integration of transcriptome, proteome and phosphoproteome data is challenging due to differences in technological methods and detection power. Hence, we first calculated the log fold change (LFC) in transcript, protein and phospho-protein abundance between KRAS-Dep and KRAS-Ind cell lines. We then correlated LFC mRNA abundance with LFC protein abundance as well as LFC protein abundance with LFC phospho-protein abundance. We found generally low to intermediate correlations, which is consistent with previous studies describing intermediate correlations between mRNA and protein abundance [22] , [23] , [24] ( Supplementary Fig. S2A,B . Correlation between LFC transcript and LFC protein 95% confidence interval (CI)=0.29–0.36, P -value 2exp-16; correlation between LFC unmodified protein and LFC phospho-protein 95% CI=0.29–0.43, P -value 2exp-16). A naive method of integrating those diverse sets of data is either to look for genes that are differentially abundant at the transcript, protein and phospho-protein level or to look for genes differentially abundant in at least one of these data sets. In this study, naive integration called 675 differentially abundant transcripts, 173 differentially abundant proteins in the unmodified state and 61 differentially abundant proteins in the phosphorylated state ( Fig. 1b and Supplementary Data 5 ). However, naive integration commonly produces a limited number of proteins that are differentially abundant across all signatures. Out of the 862 unique proteins called as differentially abundant, only 2 proteins are shared across all signatures and 45 by two independent data sets (Hochberg-adjusted P -value 0.05, Fig. 1b ) resulting in only a ~5.2% overlap among signatures. Furthermore, naive integration typically produces a final list of differentially abundant proteins that is dominated by proteins identified only in the largest data set, the transcriptome in this case ( Supplementary Fig. S2C ). Moreover, this list is enriched in genes that appear not to be causative cancer genes but that have a high dynamic range of expression ( Supplementary Fig. S2D–F ). In order to address these issues, we developed a bioinformatics methodology to integrate transcriptomics, proteomics and phosphoproteomics data sets that aims at identifying differentially abundant proteins that are nominated as such by any combination of these data sets. This methodology focuses on identifying proteins that change consistently across transcript, protein and phospho-protein levels as they constitute candidates that can be uniformly assessed, and therefore potentially used for analysing tissue samples at either the protein, phospho-protein or transcript level with similar results. We first distinguish between ‘informative’ and ‘all other’ genes and assign weights to each data set in proportion to that data set’s size ( Fig. 1a and Methods) in order to control for differences in the dynamic range of different proteins and the coverage of each ‘omics’ data set. We then calculate the combined ‘abundance score’, S , to measure the overall differential abundance of a protein across all data sets as , where z is the z -transformed LFC of protein i in the data set k , while w corresponds to the weight of each data set . N k represents the size of data set k . Our score is inspired by the Stouffer’s score that is used for meta-analysis [25] . Variations of the Stouffer score have been previously used to aggregate multiple studies involving only one type of ‘omics’ data sets, such as microarrays [26] . Moreover, although other integration methods such as the combined Fisher P -value or the scores proposed by Ramasay et al . [26] and Huang et al . [27] could be used for nominating differentially abundant proteins, when compared with those methods the S score demonstrates several key advantages for discriminating informative genes. First, because the S score normalizes the original data into z -scores, the combined distribution is also normal, allowing for simple statistics ( Supplementary Fig. S3A ). Second, the weight for each data set is flexibly defined, that is according to the size of the data set. Third, the S score can identify consistently changing proteins that would be missed otherwise ( Supplementary Fig. S3B ). Fourth, because the S score is based on the average of z i and the fisher method on the average of −log( P -value), these scores follow a close linear relationship for most values of S . Deviations of this linear relationship are observed for extreme values of S and instances where the transcript, protein and phospho-protein abundances change in discordant directions ( Supplementary Fig. S3C ). Therefore, the combined used of the Fisher and S scores could identify proteins with discordant changes in abundance. In summary, by using the S score we defined a metric for selecting transcripts, proteins and phospho-proteins that are differentially abundant uniquely or consistently across different data sets, overcoming the drawbacks of naïve integration. Our S -score analysis of the phosphoproteome, proteome and transcriptome nominated 115 differentially abundant proteins at a Hochberg-adjusted P -value 0.05. Out of the 115 proteins, 30 were nominated uniquely by our method and were missed using naive integration of the data sets ( Fig. 1c ). The S score also helps with prioritizing, as 20 proteins in phosphorylated state, 28 proteins in un-phosphorylated state and 6 transcripts that were differentially expressed would have been unattended by a naive approach ( Fig. 1c ). By using the S score, the percentage of overlap among data sets in the list of differentially expressed proteins is ~26%, which represents an increase of fivefold with respect to the naive integration approach. Moreover, genes identified by our method show higher correlation between the LFC abundance of the transcript and protein in unmodified state as well as the protein in unmodified and phosphorylated state ( Supplementary Fig. S2A,B ). We also note that the list of differentially expressed genes nominated by the S score is enriched for proteins with functions such as kinase, phospho-transferase activity and alternative splicing, and localized both in the cytoplasm and nucleus ( Supplementary Fig. S2G ). These functions are expected for proteins in signalling cascades, such as the ones downstream of KRAS, but these functions were completely missed on the proteins nominated by the naive integration approach. Finally, comparison of NSCLC KRAS-Dep cell lines against KRAS-Ind cell lines showed that of 115 proteins nominated by our integrative analysis, 68 also demonstrated increased mRNA, unmodified protein or phosphorylated protein abundance in KRAS-Dep cells, whereas 47 were found to be decreased ( Fig. 1d , Supplementary Data 6 ). Of the 68 that were increased, 57 proteins are classified as phospho-proteins, 14 as kinases, 8 as proto-oncogenes and 9 as involved in lymphocyte activation among other functions. Similarly, out of the 47 genes that were decreased, 37 are classified as phospho-proteins, 8 as kinases and 5 as proto-oncogenes among other functions. These results demonstrate that our analysis is able to identify functionally relevant proteins by integrating the transcriptome, proteome and phosphoproteome data sets. Validation in NSCLC cell lines To confirm our computational predictions, we employed a panel of 13 NSCLC cell lines for experimental studies, for which profiles of somatic mutations is provided in Supplementary Data 7 . Of these, 8 have been defined as KRAS-Ind and 5 have been defined as KRAS-Dep based on previous studies [13] , [14] and confirmed in our hands. We selected highly ranking proteins predicted to be upregulated in KRAS-Dep but not KRAS-Ind cells for further experimental validation. Of the top 20 nominated proteins, we included several proteins known to be associated with KRAS dependency in colorectal cancers (CTNNB1 and PAK1) [14] , [28] and others that have not been implicated to date (LCK and cMET) with the KRAS-Dep phenotype in any cancer ( Fig. 2 ). Western blot analyses of these proteins and their phosphorylated forms validated that cMET, LCK, PAK1 and β-catenin were enriched in expression in KRAS-Dep cell lines. Furthermore, phosphorylated forms of these proteins were also specific, suggesting that these proteins are activated in KRAS-Dep cells. These experiments validate our computational method and suggest that the S score accurately identifies proteins that are highly activated in KRAS-Dep cell lines. 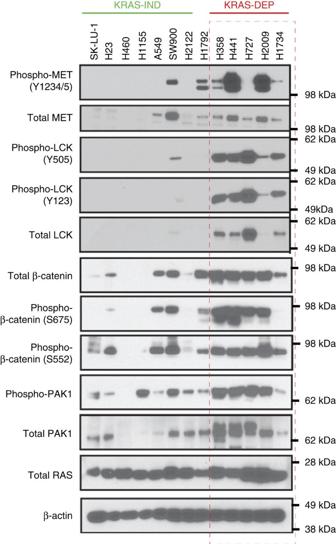Figure 2: Activation of proteins nominated by theSscore was confirmed by an orthogonal and low-throughput method. The western blot demonstrates high levels of total and phosphorylated protein forMET,LCK,PAK1and β-catenin in KRAS-Dep cells. This pattern confirms the utility of our integrative analysis in nominating differentially activate proteins. It also suggests signalling modules that are differentially active in KRAS-Dep but not in KRAS-Ind cell lines. Total RAS and β-actin were used as controls. Figure 2: Activation of proteins nominated by the S score was confirmed by an orthogonal and low-throughput method. The western blot demonstrates high levels of total and phosphorylated protein for MET , LCK , PAK1 and β-catenin in KRAS-Dep cells. This pattern confirms the utility of our integrative analysis in nominating differentially activate proteins. It also suggests signalling modules that are differentially active in KRAS-Dep but not in KRAS-Ind cell lines. Total RAS and β-actin were used as controls. Full size image Network analysis identifies active modules in KRAS-Dep cells We next developed a three-step methodology for reconstruction of biological modules associated with KRAS status ( Fig. 3a ). In the first step, we identified differential expressed pathways using the Signalling Pathway Impact Analysis algorithm (SPIA [29] ). We then build a focused undirected and weighted protein-to-protein interaction network (G). Finally, in the third step, we used the Prize Collecting Steiner Tree (PCST) algorithm to find sub-networks, T, in the weighted protein–protein interaction network (G) that maximized the number of differential expressed proteins recovered as well as the confidence in their interaction (Methods). 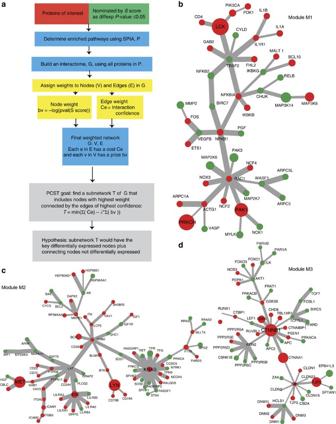Figure 3: PCST-based network reconstruction method identifies active sub-modules in KRAS-dependent cell lines. (a)Network reconstruction methodology. We built a focused undirected and weighted protein-to-protein interaction network (G) using differential expressed pathways identified by the SPIA algorithm29. We assign weights to both nodes (V) and edges (E). Node weights (bv) correspond to the −logP-value of the combined S score (S) for differential abundance between KRAS-Dep and KRAS-Ind phenotypes, whereas the edge’s (Ce) weight corresponds to the experimental confidence of that interaction as reported for the STRING database. Finally, we used the PCST algorithm to find sub-networks, T, in G that maximized the number of differential expressed proteins recovered as well as the confidence in their interaction. (b)Module M1. This module, identified by the PCST, connectsLCKandPAK1in KRAS-Dep cell lines. The module joinsLCKandPAK1with other proteins that belong to the NF-Kappa β and apoptosis pathways such asNFKBIA, NFKBs, TRAFs and BIRCs. Node size is proportional to the absolute value of the combinedSscore. Node colour represents over-expressed (red) or under-expressed (green) in KRAS-Dep cells. Edge thickness corresponds to edge’s confidence as calculated from STRING database (methods). (c)Module M2. This module, identified by the PCST, involvesKRASandMETin KRAS-Dep cell lines. Additional targetable proteins such asSYKandLYNare also part of this module. Described as inb. (d)Module M3. This module, identified by the PCST, connectsCTNNB1(β-catenin),CTNNA1,CDH1,TJP2and other proteins associated cell adhesion complexes and the tight junction pathways. Described as inb. Figure 3: PCST-based network reconstruction method identifies active sub-modules in KRAS-dependent cell lines. ( a )Network reconstruction methodology. We built a focused undirected and weighted protein-to-protein interaction network (G) using differential expressed pathways identified by the SPIA algorithm [29] . We assign weights to both nodes (V) and edges (E). Node weights (bv) correspond to the −log P -value of the combined S score (S) for differential abundance between KRAS-Dep and KRAS-Ind phenotypes, whereas the edge’s (Ce) weight corresponds to the experimental confidence of that interaction as reported for the STRING database. Finally, we used the PCST algorithm to find sub-networks, T, in G that maximized the number of differential expressed proteins recovered as well as the confidence in their interaction. ( b )Module M1. This module, identified by the PCST, connects LCK and PAK1 in KRAS-Dep cell lines. The module joins LCK and PAK1 with other proteins that belong to the NF-Kappa β and apoptosis pathways such as NFKBIA , NFKBs, TRAFs and BIRCs. Node size is proportional to the absolute value of the combined S score. Node colour represents over-expressed (red) or under-expressed (green) in KRAS-Dep cells. Edge thickness corresponds to edge’s confidence as calculated from STRING database (methods). ( c )Module M2. This module, identified by the PCST, involves KRAS and MET in KRAS-Dep cell lines. Additional targetable proteins such as SYK and LYN are also part of this module. Described as in b . ( d )Module M3. This module, identified by the PCST, connects CTNNB1 (β-catenin), CTNNA1 , CDH1 , TJP2 and other proteins associated cell adhesion complexes and the tight junction pathways. Described as in b . Full size image Specifically, in the first step we performed pathway enrichment analysis using SPIA in order to identify pathways with overall increased or decreased activity in KRAS-Dep cell lines ( Supplementary Fig. S4A ). SPIA calculates the significance of a pathway according to both a gene set over-representation index and a network’s perturbation index that takes into consideration the topology of and interactions within the pathway (Methods). This analysis revealed activation of main signalling programs in KRAS-Dep NSCLC cell lines when compared with KRAS-Ind, such as the ERBB signalling pathway, cancer-specific associated pathways and tight junctions/cell adhesion pathways ( Supplementary Fig. S4B ). Interestingly, immune-related signalling modules such as the T-cell receptor, natural killer cell-mediated cytotoxicity and Fc epsilon RI pathways were present, which suggested a relationship to LCK as immune-predominant kinase aberrantly upregulated in KRAS-Dep cells. Moreover, although cancer-associated pathways are expected to appear enriched in our analysis of cancer cell lines, it is remarkable that the cancer pathways enriched in KRAS-Dep cell lines correspond to cancers types driven by activating Ras oncogene mutations ( Supplementary Fig. S4C ), suggesting that certain molecular features are common to KRAS dependency across different cancers types. Furthermore, in the second step, we built a focused undirected and weighted protein-to-protein interaction network (G) using all proteins that belong to those pathways identified by SPIA and we assigned weights to both nodes (V) and edges (E). The weight of each Node (bv) corresponds to the −log P -value of the combined score ( S ) for differential abundance between KRAS-Dep and KRAS-Ind phenotypes, whereas the weight of each edge (Ce) corresponds to the experimental confidence on that interaction. The edge weight is derived from the STRING database [30] by combining STRING’s experimental and physical interaction scores using a naive Bayesian approach. Finally, in the third broad step of this methodology, in order to identify specific network sub-modules that are active in KRAS-Dep cell lines, we formulated this network reconstruction task as a PCST problem [27] , [31] , [32] , [33] (Methods). The PCST allowed us to synthesize transcriptome, proteome and phosphoproteome signatures in the context of the weighted protein-to-protein interaction network mentioned above. This formulation facilitated the identification of crosstalk between pathways nominated by SPIA, as well as identification of relevant proteins that were not directly measured in our experiments. We identified three modules—referred to as M1, M2, M3—using the PCST formulation. M1 contains LCK, PAK1 and PRKCH as well as proteins involved in the regulation of inflammation, antiviral responses and apoptosis proteins such as several TRAFs, BIRCs and NFKBs ( Fig. 3b ). M2 contains KRAS as well as the kinases MET, LYN, SYK and MAPK1 among others ( Fig. 3c ). M3 contains CTNNB1 (β-catenin), CDH1, CTNNA1 (α-catenin), TJP2 and other proteins associated with the adhesion complex ( Fig. 3d ). M3 is consistent with our observation that β-catenin is mainly localized in the cellular membrane of KRAS-Dep cells ( Supplementary Fig. S4D ), supporting a role in cellular adhesion in NSCLC cell lines. KRAS–LCK–PAK1 signalling axis in KRAS-Dep lung cancer Intriguingly, module M1 suggests a link between LCK and PAK1 that has not been reported previously in solid tumours despite the fact that PAK1 overexpression has been already implicated in lung and breast cancers [34] . LCK is a tissue-specific kinase normally expressed in T-lymphocytes. It is commonly overexpressed in myeloid and lymphocytic leukaemia, as well as Burkitt and non-Hodgkin’s B-cell lymphoma [35] and acts as a proto-oncogene, inducing cellular transformation through the regulation of cell proliferation and survival [35] , [36] . A role for LCK is not known in solid tumours. Therefore, we hypothesized that the aberrant overexpression of LCK in KRAS-Dep lung cancers could also have a role in this disease. To confirm our network reconstruction approach and further dissect the functional connections among KRAS, MET and LCK, we performed knockdown experiments using independent siRNAs in the H441 and H358 cell lines that display KRAS dependency [13] . Immunoblot analysis showed that knockdown of KRAS decreased the abundance of MET, phospho-MET, LCK, phospho-LCK, phospho-PAK1/2 and phospho-BAD ( Fig. 4a ; Supplementary Fig. S5A,B ). These results demonstrate that MET, LCK, PAK1/2 and BAD are downstream of KRAS and regulated by KRAS in vitro . In contrast, knockdown of LCK did not reduce KRAS levels, indicating that LCK does not regulate KRAS protein abundance ( Fig. 4b , Supplementary Fig. S5C ), although previous reports have suggested a role for LCK in KRAS activation [37] . Knockdown of LCK did however reduce phospho-PAK1/2 levels but not total PAK1/2 protein, defining PAK1/2 as targets for LCK-mediated phosphorylation ( Fig. 4b ; Supplementary Fig. S5C ). Figure 3b indicates that this effect is potentially mediated through a small network of interacting proteins. Moreover, knockdown of PAK1/2 did not change the phosphorylation or protein levels of LCK, confirming that PAK1 and PAK2 are downstream of LCK ( Fig. 4c ). Taken together, our bioinformatics and experimental results suggest an active KRAS–LCK–PAK1/2 network in KRAS-Dep cell lines ( Supplementary Fig. S5D ). Our results also present evidence that KRAS can influence both the phosphorylation and protein levels of LCK and MET kinases, which complements previous reports suggesting that those kinases could be upstream of the RAS-MEK pathways [37] , [38] , and suggests the possibility of a feedback loop among these proteins in KRAS-Dep cells ( Supplementary Fig. S5D ). 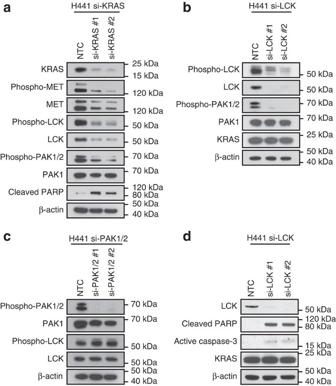Figure 4: Experimental validation of protein modules in KRAS-Dep cells. (a)KRASinfluences total and phosphorylated protein level of potential druggable kinasesLCKandMETin KRAS-Dep cell lines. Knockdown ofKRASwith two independent siRNAs reduces phosphorylation levels ofLCK,MET,PAK1/2in H441 cell line. KRAS-KD also reduced total protein levels ofLCKandMETbut notPAK1/2. (b)LCKinfluencesPAK1/PAK2activation in KRAS-Dep cell lines. Knockdown ofLCKusing two independent siRNAs reduces phosphorylation levels of PAK1/2 but not their protein level in H441 KRAS-Dep cell line. (c)PAK1/2are downstream of LCK in KRAS-Dep cell lines.PAK1/2knockdown does not affect phosphorylation or protein level ofLCKin H441-Dep cell line. (d)LCKknockdown increases the level of cleavedPARPand caspase-3, markers of apoptosis in H441 KRAS-Dep cell line. Figure 4: Experimental validation of protein modules in KRAS-Dep cells. ( a ) KRAS influences total and phosphorylated protein level of potential druggable kinases LCK and MET in KRAS-Dep cell lines. Knockdown of KRAS with two independent siRNAs reduces phosphorylation levels of LCK , MET , PAK1/2 in H441 cell line. KRAS-KD also reduced total protein levels of LCK and MET but not PAK1/2 . ( b ) LCK influences PAK1/PAK2 activation in KRAS-Dep cell lines. Knockdown of LCK using two independent siRNAs reduces phosphorylation levels of PAK1/2 but not their protein level in H441 KRAS-Dep cell line. ( c ) PAK1/2 are downstream of LCK in KRAS-Dep cell lines. PAK1/2 knockdown does not affect phosphorylation or protein level of LCK in H441-Dep cell line. ( d ) LCK knockdown increases the level of cleaved PARP and caspase-3, markers of apoptosis in H441 KRAS-Dep cell line. Full size image KRAS-Dep cells are also dependent on LCK for proliferation In order to extend our results and investigate potentially aberrant expression of LCK in other cell lines, we performed a gene outlier expression analysis on an extended panel of 122 lung cancer cell lines (11 KRAS-Dep, 18 KRAS-Ind and 93 KRAS-WT) (Methods). We evaluated informative genes observed as outliers in KRAS-Dep but not in KRAS-Ind cell lines ( Fig. 5a ). 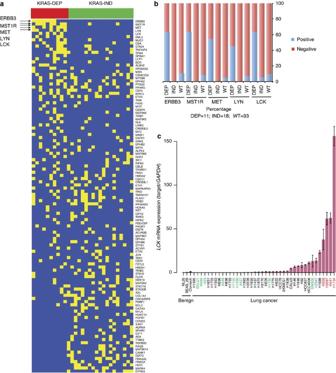Figure 5: Outlying kinases in KRAS-Dep cell lines. (a) Cancer outlier profile analysis (COPA) of ‘informative’ genes on an extended gene expression data set of KRAS-mutated cell lines confirmsLCK,MET,LYNandERBB3as differentially abundant proteins in KRAS-Dep but not in KRAS-Ind cell lines. Eleven KRAS-Dep and 18 KRAS-Ind were analysed. (b) OverexpressedLCKis present in at least 60% but in <10% of the either wild type or KRAS-Ind cell lines.MET,ERBB3,MST1RandLYNshow a similar pattern. 11 KRAS-Dep, 18 KRAS-Ind and 93 KRAS-WT cell lines were analysed. (c)LCKexpression measured by QRT–PCR in a panel of KRAS-Dep (red label), KRAS-Ind (green label) and KRAS-WT (black label) cell lines confirms high levels ofLCKin KRAS-Dep cell lines and none or negligible expression in KRAS-Ind or WT cell lines. Cell line H2347 (blue label) harboursNRASQ61K mutation, but its dependency status could not be established. Bar height corresponds to the average over three independent replicates and error bars are defined as s.e.m. Figure 5: Outlying kinases in KRAS-Dep cell lines. ( a ) Cancer outlier profile analysis (COPA) of ‘informative’ genes on an extended gene expression data set of KRAS-mutated cell lines confirms LCK , MET , LYN and ERBB3 as differentially abundant proteins in KRAS-Dep but not in KRAS-Ind cell lines. Eleven KRAS-Dep and 18 KRAS-Ind were analysed. ( b ) Overexpressed LCK is present in at least 60% but in <10% of the either wild type or KRAS-Ind cell lines. MET , ERBB3 , MST1R and LYN show a similar pattern. 11 KRAS-Dep, 18 KRAS-Ind and 93 KRAS-WT cell lines were analysed. ( c ) LCK expression measured by QRT–PCR in a panel of KRAS-Dep (red label), KRAS-Ind (green label) and KRAS-WT (black label) cell lines confirms high levels of LCK in KRAS-Dep cell lines and none or negligible expression in KRAS-Ind or WT cell lines. Cell line H2347 (blue label) harbours NRAS Q61K mutation, but its dependency status could not be established. Bar height corresponds to the average over three independent replicates and error bars are defined as s.e.m. Full size image This analysis revealed LCK, MET, ERBB3, MST1R and LYN are kinases that frequently exhibit outlier expression in KRAS-Dep cell lines, with expression levels in the top 80 percentile in >60% of cell lines in this group ( Fig. 5b ). By contrast, the kinases DYRK4 and MARK4 showed outlier expression in KRAS-Ind cell lines ( Fig. 5a ). To validate our approach, we experimentally confirmed that LCK is overexpressed in KRAS-Dep cells using quantitative PCR on a panel of 43 lung cell lines ( Fig. 5c ). Given that LCK is a known lineage-specific proliferation factor in B lymphocytes, we hypothesized that KRAS-Dep NSCLC overexpressing LCK also require this kinase for cell growth and survival. We performed shRNA knockdown experiments for LCK and determined whether ablation of LCK activity with independent shRNAs could selectively impair cell proliferation on KRAS-Dep cells (Methods). 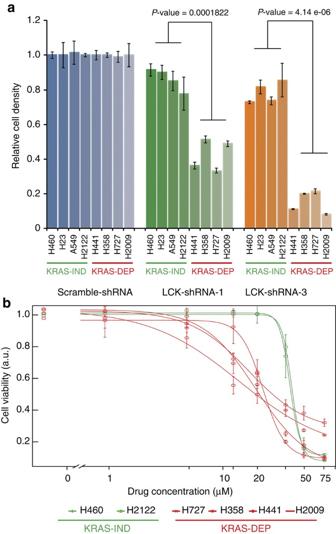Figure 6:LCKconstitutes a potential novel drug target in NSCLC KRAS-Dep cell lines. (a)LCKknockdown impairs cell proliferation specifically in KRAS-Dep cell lines.LCKknockdown with two independent shRNAs showed statistically significant reduction in cell proliferation in KRAS-Dep but not KRAS-Ind cell lines (LCKshRNA-1t-testP-value=0.0001822 andLCKshRNA-3t-testP-value=4.14 exp−06). Bars correspond to the average of three independent experiments and error bars are defined as s.e.m. (b) Inhibition ofLCKusing small-molecule inhibitor preferentially impaired cell proliferation in KRAS-Dep but not in KRAS-Ind cell lines. Points represent the average over four independent experiments and error bars are defined as s.e.m. Figure 6a shows that knockdown of LCK dramatically impairs cell proliferation in KRAS-Dep cells but not KRAS-Ind cells, validating our predictions (shRNA1 t -test P -value=0.0001822, shRNA3 t -test P -value=4.14 exp −6). We further confirmed that independent knockdown of KRAS also produced similar results ( Supplementary Fig. S6A ). Figure 6: LCK constitutes a potential novel drug target in NSCLC KRAS-Dep cell lines. ( a ) LCK knockdown impairs cell proliferation specifically in KRAS-Dep cell lines. LCK knockdown with two independent shRNAs showed statistically significant reduction in cell proliferation in KRAS-Dep but not KRAS-Ind cell lines ( LCK shRNA-1 t -test P -value=0.0001822 and LCK shRNA-3 t -test P -value=4.14 exp−06). Bars correspond to the average of three independent experiments and error bars are defined as s.e.m. ( b ) Inhibition of LCK using small-molecule inhibitor preferentially impaired cell proliferation in KRAS-Dep but not in KRAS-Ind cell lines. Points represent the average over four independent experiments and error bars are defined as s.e.m. Full size image Moreover, as a kinase, LCK is also an attractive candidate for strategies of targeted therapy. While specific LCK inhibitors are still in development, we tested whether prototype small molecule inhibitors of LCK would selectively affect the viability of NSCLC KRAS-Dep cells. We treated a panel of 3 KRAS-Dep cell lines and 2 KRAS-Ind cell lines with increasing doses of LCK inhibitor (CAS 213743-31-8) and measured cell viability at different drug concentrations. All three KRAS-Dep cell lines tested in this experiment were sensitive to LCK inhibition, whereas the KRAS-Ind cell lines were insensitive to LCK inhibition, as expected from our hypothesis ( Fig. 6b ). We further confirmed these results using a second LCK inhibitor (CAS 918870-43-6) that showed similar results ( Supplementary Fig. S6B ). These results demonstrate that KRAS-Dep lung cancer cell lines have aberrant overexpression and activity of LCK. Similarly, we observed that MET shRNA knockdown as well as MET inhibition with small molecule inhibitors selectively impaired cell growth of KRAS-Dep cell lines ( Supplementary Fig. S6C,D ), further supporting the biological relevance of our computational network reconstructions and predictions of targetable proteins in KRAS-Dep cells. To evaluate whether LCK expression can be used to stratify the KRAS dependency status of human lung cancers, we assessed LCK expression in a panel of 29 lung adenocarcinoma tissue samples with mutations in KRAS. To confirm the KRAS mutations, we genotyped canonical positions in codons 12, 13 and 61, known to produce a constitutively active KRAS when mutated ( Supplementary Table S1 ). As there is currently no clinical biomarker to identify the KRAS dependency status of NSCLCs, we sought to evaluate LCK expression in these samples as a potential biomarker for KRAS dependency. As LCK is normally highly expressed in lymphocytes, LCK mRNA expression from surgical samples is not an accurate method to assess LCK expression in epithelial-derived lung cancer cells, as the infiltrating lymphocytes in these samples would distort the analysis. Thus, a previous study that detected LCK in lung cancer tissues by gene expression microarrays is likely confounded by the lack of cell-type specificity [39] . We therefore used immunohistochemistry (IHC) to determine the abundance of phosphorylated LCK in epithelial lung cancer cells in our 29 clinical samples. We first validated our IHC assay using a panel of normal tissues and cell lines that demonstrated high levels of LCK expression in the spleen where lymphocytes are abundant, but not in other tissue types. Next, a TMA of KRAS-Dep cell lines H441 and H358 also showed high levels of phosphorylated LCK expression, whereas a TMA of H460 and H23 KRAS-Ind cell lines did not showed any staining. Finally, applying this method to our 29 lung tumour samples harbouring KRAS mutation, we found that 58.6% (17/29) of tumours showed high levels of phosphorylated LCK staining, whereas 41.4% (12/29) tumours showed low levels of phosphorylated LCK ( Supplementary Table S1 ). These results are consistent with in vitro data demonstrating that KRAS-mutant lung cancer tissues can be subdivided in two groups according to their levels of phosphorylated LCK, similar to NSCLC cell lines. Although, it is not possible currently to determine the dependency status of a tissue through direct experimentation, this subdivision of tumour samples is suggestive of the correlation described here between KRAS dependency and LCK activation in cell lines. However, a larger cohort of tissues with matched profiles of KRAS mutation, gene expression as well as IHC of phosphorylated LCK would be required to further determine the prognostic value and the extent of this association between KRAS dependency and LCK activation in tissue specimens. A proof-of-principle analysis in this direction is shown in Supplementary Fig. S6E . KRAS and LCK could regulate anti-apoptosis pathways To explore potential functional roles of the KRAS–LCK–PAK1/2 pathway, we evaluated our computational predictions of modules M1, M2, and M3 in lung cancer. We were struck by the enrichment for apoptosis-related proteins in module M1 that included LCK and PAK1 ( Supplementary Fig. S7A ), suggesting a potential connection between LCK and apoptosis. Indeed knockdown of LCK in H441 cells was correlated with increased levels of cleaved PARP and caspase-3, markers of apoptosis, which further supports the association between LCK and apoptosis ( Fig. 4d ). To further explore this association, we used microarrays to profile gene expression changes following knockdown of LCK in the H441 and H358 KRAS-Dep cell lines, and we evaluated the microarray data for pathways specifically inhibited or activated by LCK ( Supplementary Table S2 and Methods for specific details on this analysis of these microarray data). We assumed that pathways activated specifically by LCK in the context of KRAS dependency would be inhibited after knockdown of this kinase. Interestingly, we observed a module composed of TRAF1, BIRC3 and BCL2L1, three proteins that regulate apoptosis ( Supplementary Fig. S7B ). These proteins were part of a canonical KEGG pathway for lung small cell cancer, a pathway specifically inhibited after LCK knockdown ( Supplementary Table S2 ). Moreover, we reasoned that causative genes should be both overexpressed in KRAS-Dep compared with KRAS-Ind cell lines and also downregulated upon LCK knockdown in H441 and H358 (Methods). Performing this analysis yielded BCL2A1, a BCL2-related protein A1 ( Supplementary Fig. S8A,B ). BCL2A1 can bind to and inhibit or neutralize pro-apoptotic multi-domain proteins such as BAK and BAX as well as pro-apoptotic BH3-only proteins such as tBID, BIM, PUMA, BIK, HRK and NOXA but not BAD [40] . Pro-apoptotic protein BAD is inhibited when phosphorylated [41] , [42] . Indeed, knockdown of KRAS in H441 decreased phosphorylation levels of BAD (p112, p136) ( Supplementary Fig. S5A ), which is consistent with increased levels of cleaved PARP observed in the knockdown samples ( Fig. 4a ) and supports a role for KRAS in preventing apoptosis via BAD. The effect on BAD phosphorylation was observed downstream of KRAS but not downstream of LCK or PAK1/2. Knockdown of LCK or PAK1/2 did not decrease phosphorylation levels of BAD, suggesting independent mechanisms. Taken together, these computational and experimental data suggest a potential regulatory network in KRAS-Dep cells that both ‘directly’ inhibits apoptosis by inducing phosphorylation of BAD and ‘indirectly’ by modulating the apoptotic response through the LCK module. The advent of high-throughput technologies has greatly advanced the study of cancer biology. However to date, most studies employ only an individual technology and studies that do include multiple profiling technologies frequently analyse them separately without integrating across modalities. While these approaches are effective for identifying single events in cancer (that is, a new point mutation or an overexpressed gene), they do not uncover integrated biological modules that coordinate higher-level biological processes (that is apoptosis, RNA splicing, and so on). Here we developed a novel method to integrate disparate profiling modalities to explore novel functional networks differentiating KRAS-Dep from KRAS-Ind NSCLCs. We used transcriptome, proteome and phosphoproteome profiling to comprehensively analyse gene expression at the RNA and/or protein level, as well as signalling proteins activated or inactivated by post-translational modification. Using this approach on 13 KRAS-mutant NSCLC cell lines known to be KRAS-Dep or KRAS-Ind, our integrative analysis nominated 115 proteins that were differentially abundant between these two groups (Hochberg-adjusted P -value 0.05). Specifically, our method identified a set of proteins with highly correlated changes between transcript and protein levels or unmodified protein and phosphorylated protein levels, and then enriched these results for specific functions associated with KRAS. Of these, we validated four proteins (LCK, MET, PAK1 and β-catenin) selected from the top 20 nominated genes. LCK, MET and PAK1 have not previously been studied in the context of KRAS-Dep lung cancer. Of particular interest to this study was LCK, a lymphocyte-specific kinase well studied in B-lymphocyte development [35] , [36] but uncharacterized in solid tumours. We define a KRAS–LCK–PAK1/2 pathway in KRAS-Dep lung cancers that has not previously been described. We find that KRAS regulates LCK protein and phospho-protein levels, and LCK in turn regulates PAK1/2 phosphorylation but not total protein levels. Previous studies have identified a role for PAK1/2 in the phosphorylation of β-catenin in KRAS-mutated colorectal cancer [14] , [28] ; however, we did not observe β-catenin as a direct target of the KRAS–LCK–PAK1/2 pathway in lung cancer. Knockdown of KRAS and LCK did not impact β-catenin phosphorylation or cellular localization. Indeed β-catenin localized to the cell membrane in our experiments ( Supplementary Fig. S4D ), not to the cell nucleus where β-catenin is known to be active in the stimulation of the Wnt signalling pathway [14] , [28] . In addition, our work finds that β-catenin associates with the M3 reconstructed network module that also contains cell surface adhesion proteins such as CDH1, CTNNA1 (α-catenin) and TJP2. Thus β-catenin in NSCLC cell lines may operate through cell adhesion pathways as opposed to a role in regulating transcription, as reported in colorectal cancer [14] . This further helps to explain earlier observations that associate KRAS-Dep lung cancer cell lines with differentiated phenotypes [13] . To explore the function of LCK in lung cancer, we performed knockdown experiments and observed that depletion of LCK impaired cellular proliferation and phenocopied knockdown of KRAS in KRAS-Dep cell lines. In addition, small-molecule inhibition of LCK resulted in preferential decrease in cell viability in KRAS-Dep cells. Using the PCST formulation, we also found that LCK was associated with a reconstructed Module M1 containing several proteins involved in the regulation of apoptosis in addition to PAK1. Indeed, we observed that knockdown of LCK or KRAS induce an increase in cleaved PARP levels, indicating an increase in apoptosis. KRAS-Dep cells may then modulate apoptosis through two complementary mechanisms. KRAS may regulate the apoptotic response by regulating phosphorylation of BAD, whereas LCK may regulate BCL2-related anti-apoptotic proteins. Previous studies in T cells and CLL cells support this role of LCK as a guardian against apoptosis, as well as LCK inhibition through small-molecule inhibitors as an effective mean to sensitize those cells to apoptosis [35] . Finally, we evaluated LCK expression in KRAS-mutant NSCLC tumours. We observed that ~60% (17/29) of the KRAS-mutated tumours showed high staining levels of phosphorylated LCK by IHC, suggesting that they are probably KRAS-Dep. As projects such as The Cancer Genome Atlas (TCGA) approach their goal of enrolling thousands of patients with matched omics data sets such as exome/genome and RNA sequencing and reverse-phase protein arrays (among others), as well as detailed clinical follow-ups, we will be able to assess the prognostic value of the LCK-KRAS-PAK1/2 pathway in the context of KRAS dependency. A proof-of-principle analysis in this direction is presented in Supplementary Fig. S6E . Taken together, this study establishes a potentially actionable pathway in KRAS-Dep NSCLCs comprising KRAS, LCK and PAK1/2. We find that KRAS induces LCK activation, leading to a signalling cascade specific to KRAS-Dep cells that promotes cell proliferation and could reinforce a positive feedback loop with KRAS activity ( Supplementary Fig. S5D ). Furthermore, our study develops a method to integrate multiple proteomic and transcriptomic data sets for the identification of biologically relevant modules in cancer. We thus provide a framework for the complex analysis of multiple cancer data sets to make biologically informed computational predictions for uncharacterized signalling pathways in cancer. Data used in this study A summary of the data sets and software used in this study is provided in Supplementary Table S3 . Protein quantification by label-free LC-MS/MS The mass spectrometry proteomics and phosphoproteomics data have been deposited to the ProteomeXchange Consortium ( http://proteomecentral.proteomexchange.org ) via the PRIDE partner repository [43] with the data set identifier PXD000439. The general workflow used for label-free phosphoproteome quantification is summarized in the following steps [18] , [44] , [45] , [46] , [47] , [48] , [49] , [50] , [51] , [52] , [53] , [54] , [55] , [56] , [57] , [58] : sample preparation, phospho-peptides enrichment, label-free quantitative tandem mass spectrometry, peptide identification through database search and quantification by the spectral count method. Cell lines were grown on manufacturer-recommended media until they were 70% confluent and then protein extraction and sample preparation were performed, as previously reported [18] , in the presence of proteases and phosphatases. For mass spectrometry, eluted proteins were separated by one-dimensional (1D) SDS–PAGE (4–12% Bis-Tris Novex-Invitrogen, Carlsbad, CA, USA). Twenty four equal-sized gel bands were excised and subjected to in-gel tryptic digestion. As phospho-peptides correspond to a small fraction of all peptides after tryptic digestion, phospho-peptide enrichment was performed using immobilized metal affinity chromatography (IMAC). Tryptic peptides were then divided into two fractions: phospho-enriched and flow-through or unmodified peptides. Both fractions of extracted peptides were independently reconstituted with mobile phase A prior to on-line reverse phase nanoLC-MS/MS (LTQ-Velos with Proxeon nanoHPLC, ThermoFinnigan). Peptides were eluted on-line to the mass spectrometer with a reverse phase linear gradient from 97% A (0.1% formic acid in water) to 45% B (0.1% formic acid in acetonitrile) over 60 min. Peptides were detected and fragmented in the mass spectrometer in a data-dependent manner, sending the top 12 precursor ions that exceeded a threshold of 500 ion counts, excluding singly charged ions, for collisional-induced dissociation. Dynamic mass exclusion was enabled with a repeat count of 2 for 1.5 min for a list size of 500 m/z . For the database search, raw spectra files were converted to mzXML using ReadAW. The mzXML files were searched using X!Tandem with the k -score plug-in [59] . The proteomic searches were performed using the following options: allow up to two missed tryptic cleavages, a parent ion tolerance window of −1 to +4 Da and a fragment ion tolerance of 0.8 Da. The following variable modifications were allowed: phosphorylation of serine, threonine and tyrosine (+79.966331@(STY)), oxidation of Methionine (+15.994920@M) and carbamidomethylation of Cysteine (+57.021460@C). All protein searches were performed using the Human Refseq protein database (release 47). Appended to this database were common proteomic contaminants and reversed protein sequences to serve as decoys [60] , [61] . The X!Tandem results were then post-processed with PeptideProphet and ProteinProphet [62] , [63] . Spectral counts were then obtained for all of the proteins identified in our cohort of 13 cell lines using the Abacus software tool [64] . For Abacus, the following parameters were used: count only peptide-to-spectrum-matches with a PeptideProphet score of >0.5 (iniProbTH=0.50), retain only proteins with at least one peptide with a PeptideProphet score of >0.99 (maxIniProbTH=0.99) and a ProteinProphet probability of >0.9 in the COMBINED file (minCombinedFilePw=0.90). For the phosphorylated fraction, peptides were required to have at least one phosphorylated serine, threonine or tyrosine (reqAAmods=+S[167];+T[181];+Y[243]). Proteins and phospho-proteins identified with at least one spectral count in two independent cell lines were kept for downstream analysis ( Supplementary Data 1 and 3 ), whereas those identified in one cell line only were filtered out ( Supplementary Data 2 and 4 ). The spectrum counts for each protein were normalized with respect to the total number of spectrum counts within each sample. This normalization was applied independently for unmodified and modified proteins. Common contaminants and ‘Deja vu’ [65] proteins were filtered out before quantification of differentially abundant proteins. For both unmodified and phosphorylated proteins the fold change was calculated with respect to the comparison KRAS-Dep versus KRAS-Ind cell lines. This fold change was then log-transformed and z -score-normalized. Finally, the P -value was calculated using the standard normal distribution. The final master tables with the normalized spectrum counts for phosphorylated and flow through fraction for each cell line are provided as Supplementary Data 1 and 2 . Phospho-enrichment was calculated as the ratio between the number of phospho-peptides identified and the total number of peptides (phosphorylated and unphosphorylated) at a particular PeptideProphet score for the best peptide match (bestInitProbability). All enrichment calculations were made using only peptides that have Ser, Thr or Tyr in them. Peptides without any of those amino acids were excluded from the calculation. Finally, the phospho-enrichment value is taken for a PeptideProphet score of >0.94 (bestInitProbability=0.9413), which produces a 0.01 FDR. The calculated phospho-peptide enrichment, for all samples, ranges from 26 to 38%. Gene expression data Gene expression data used in this study are publicly available at ArrayExpress with accession number E-MTAB-783 . Gene expression was scaled and log2-normalized before additional downstream analysis. Integration of data sets As different protein functional groups (for example, transcription factors, kinases or secretory proteins) have distinct gene expression dynamic range, the gene expression data set was split into two different categories, ‘informative’ genes and ‘all other’ genes and subsequently analysis were performed independently on each one of them. ‘Informative’ refer to genes that are well known to drive a carcinogenic process such as KRAS , TP53 , ERBB2 and CDKN2A , and so on, as well as to genes that could have the potential to drive oncogenesis as kinases, phosphatases among others. A list of ‘Informative’ genes was compiled by combining the Sanger’s cancer census genes, all kinases and phosphatases as well as additional and recently reported genes important for carcinogenesis ( Supplementary Data 8 ). Raw data was preprocessed as described above. Phosphoproteome, proteome and transcriptome data sets were log-transformed and the LFC was taken with respect to the comparison between KRAS-Dep and KRAS-Ind cell lines. The LFC was z -score-normalized and a P -value was calculated using the standard normal distribution. In order to synthetize for each protein the information obtained from gene expression, protein and phospho-protein abundance, we calculated a combined abundance S score as , where z is the z -transformed LFC of protein i in the data set k , whereas w corresponds to the weight of each data set . N k represents the size of data set k . Finally, a P -value for the combined score was calculated using the standard normal distribution and then adjusted using Hochberg procedure in order to correct for multiple hypothesis testing. Network analysis We use SPIA [29] in order to perform network-enrichment analysis. The source code for this algorithm is available as an R package from http://bioconductor.org/biocLite.R . SPIA calculates the significance of a pathway according to both the over-representation evidence (for example, any commonly used enrichment test) and perturbation-based evidence using the topology of the network. The KEGG database ( http://www.genome.jp/kegg/kegg1.html ) was used as the main source for the pathway’s definition and we used the set of differentially expressed genes as defined by the combined abundance score with adjusted P -value 0.05 as the seed genelist. Significant pathways with FDR 0.05 are reported ( Supplementary Table S4 ). For the Network reconstruction methodology, we build a focused undirected and weighted protein-to-protein interaction network (G) using significant (FDR 0.05) pathways identified by SPIA [29] . Those pathways were downloaded from the KEGG database [66] and then merged into a unified meta-pathway (G) using the bioconductor KEGGgraph library [67] . This meta-pathway (G) is provided for the interested reader as Supplementary Data 9 . We assigned weights to both nodes (V) and edges (E). Node weights correspond to the combined score ( S ) for differential abundance between KRAS-Dep and KRAS-Ind phenotypes, whereas the edge weights correspond to the experimental confidence on that interaction as derived from the STRING database. For each edge in the meta-pathway, we obtained from STRING the experimental and physical interaction scores and then combined them into a single score using a naive Bayes approach. In addition, in order to decrease redundancy, multiple gene family members with the same interaction partners were summarized into a ‘consensus gene’ defined as the gene with highest scoring interaction neighbourhood. This step is advised due to the node redundancy introduced within the KEGG database and the fact that the interactions for many gene family members are annotated by similarity to other members in the family and not by direct experimental validation. Finally, we used PCST algorithm to find sub-networks, T, in the meta-pathway (G) that represent the most differentially abundant proteins connected through the most reliable interactions. Formally, the PCST is formulated as follows: where b v =−log p ( S ) with p ( S ) as the P -value for the S score of each protein, and with R i for the string score for the edge’s physical and experimental evidence. This choice of b v and c e assigns high values to the most differentially abundant proteins in the pathway and low values to the high confidence interactions in the network. Finally, the constant λ controls the trade-off of adding new proteins into the reconstructed network, by balancing the cost of new edges and the prize gained by bringing in a new protein. λ indirectly controls the size of the final sub-networks. All results presented here were obtained with λ =0.3. In order to choose λ , we solved the PCST problem, varying λ between 0.01–1 in increments of 0.01, and choose the value of λ at which 60% of the essential nodes of simulated network of similar size were recovered. In order to solve the PCST, we used the implementation based on information message passaging described by Bailly-Bechet et al . [33] , for which the source code availability is annotated in the Supplementary Table S3 . The PCST has been used in similar settings before [27] , [32] , [33] because it identifies sub-networks that represent cross-talk between pathways, as well as ‘connecting proteins’ that are not directly measured in the experiment but that are relevant to link other measured proteins with high weight in the network. Analysis of LCK knock-down experiments We used SPIA as described above to identify pathways specifically activated or inhibited after LCK knockdown ( Supplementary Table S2 ), confirming the involvement of a lung cancer pathway but more importantly several pathways controlling apoptosis induction such as the natural killer cell-mediated cytotoxicity, Toll-like receptor signalling and the NOD-like receptor signalling pathway. This is in agreement with the fact that Module M1 containing LCK and PAK1 were enriched for proteins belonging to the apoptosis pathways ( Supplementary Fig. S7A ). Therefore, we focused the additional analysis of the microarray data on identifying altered proteins belonging to the apoptosis pathways. To perform BCL2A1 nomination we first collect apoptosis gene concepts from KEGG, gene ontology and Reactome and generate a meta-apoptosis gene concept with all unique genes found. We reasoned that proteins specifically activated by LCK should simultaneously satisfy the following three characteristics: to be overexpressed when comparing KRAS-Dep versus KRAS-Ind cells, to be under-expressed when comparing the LCK knock down versus the non-targeting control in H441 and H358 cell lines and to be unaffected after knocking down any other gene in different cell lines. Characteristic 3 is included to control for changes in gene expression induced by any knockdown treatment irrespective of the gene of interest. Representing conditions 1, 2 and 3 in Cartesian coordinates results in a plot shown in Supplementary Fig. S8A . The x axis shows the differential expression of those genes when comparing KRAS-Dep versus KRAS-Ind cell lines. The y axis shows the average differential expression of the same genes when comparing a siRNA knockdown of LCK in H441 and H358 cell lines with respect to the targeting control (red dots), or the average differential expression when comparing the knockdown of a ‘random’ gene compared to its respective control (black dots) in three unrelated prostate cell lines. Genes affected by the overall siRNA treatment would be overlapping or very close in this plot, whereas genes specifically affect by LCK would be located far apart in the y axis. We measure this effect by taking the Euclidean distance between red and black dots representing the same gene in the above representation. Genes that are specifically affected by LCK would have positive or negative Euclidean distances according to the magnitude of their perturbation, whereas genes nonspecifically affected by the siRNA treatment would have Euclidean distances close to 0 ( Supplementary Fig. S8B ). Cell lines All cell lines were obtained from ATCC and maintained using standard procedures. Specifically, H441, H358, H2009, H1734, H727, H460, H2122, H1792, H23 and H1155 cells were maintained in RPMI 1640 (Gibco) plus 10% FBS and 1% penicillin-streptomycin. A549 cells were maintained in DMEM (Gibco) plus 10% FBS and 1% penicillin–streptomycin. SKLU1 cell were maintained in DMEM/F12 plus 10% FBS and 1% penicillin–streptomycin. SW900 cells were maintained in L15 plus 10% FBS and 1% penicillin–streptomycin. Cell lines were grown at 37 °C in a 5% CO 2 cell culture incubator. All cell lines were genotyped for identity at the University of Michigan Sequencing Core. shRNA knockdown studies For LCK and KRAS knockdowns, all cells were plated at 100,000 cells per ml in six-well plates and allowed to attach overnight. Cells were infected the following day with the lentivirus RNA and 24 h after infection old media was replaced with new cell media. Cells were allowed to grow for 96 h in this fresh media. At this point cells were treated with 1 mg ml −1 puromycin for 5 days to eliminate uninfected cells. Media was replaced and proliferation assays set up with the stable selected clones. Knockdown efficiency was confirmed by western blot. shRNA sequences are provided in the Supplementary methods . siRNA knockdown studies Cells were plated in 100-mM plates at 30% confluency and transfected twice at 12 h and 24 h post-plating. Knockdowns were performed using 20 uM siRNA oligos or non-targeting controls (Dharmacon) with Oligofectamine (Invitrogen) in Opti-MEM media (Gibco). Knockdown efficiency was confirmed by western blot. siRNA used are listed in the Supplementary methods . Seventy-two hours post transfection, cells were rinsed twice with 10 ml PBS, harvested with a rubber policeman in 1 ml PBS and centrifuged for 5 min at 2,500 g . The supernatant was discarded and the cells were prepared for western blot analysis. Western blots Cell pellets were lysed in RIPA lysis buffer (Sigma) supplemented with HALT protease inhibitor and phosphatase inhibitor (Fisher). Western blotting was performed using standard protocols. Briefly, protein lysates were boiled in sample buffer for 5 min at 98C and 10 ug of protein was separated by SDS–PAGE gel electrophoresis. Proteins were transferred onto a PVDF membrane (GE Healthcare) and blocked for 30 min in blocking buffer (5% milk in 1 × TBS supplemented with 0.1% Tween (TBS-T)). Membranes were incubated with primary antibody overnight at 4 °C and then with secondary antibody for 2 h at room temperature. Signals were visualized by enhanced chemiluminescence system (GE Healthcare). The primary antibodies used are listed in the Supplementary methods and full blots can be found in Supplementary Fig S9–S15 . Proliferation assays Proliferation assays were performed with stable clones of the scramble RNA, and two independent constructs against LCK or KRAS for each cell line. Cells were plated at 30,000 cells per ml in 24-well plates and cell counts were taken with a Beckman coulter Z2 particle-count instrument every 48 h for 8 days. Three independent replicates of each experiment were performed. WST drug assays Cells were plated in a 96-well plate 12 h prior to drug treatment at a density of 3,500 cells per well in 100 ul of growth media. Desired concentrations of LCK Inhibitor (Santa Cruz, sc-204052, CAS 213743-31-8) and LCK Inhibitor II (Millipore, Lck Inhibitor II, CAS 918870-43-6) were prepared using growth media and 100 ul of the drug solution was added directly to the wells. After 72 h of incubation at 37C, 20 ul of WST Cell proliferation reagent (Roche) was added to each well. Following 2 h of incubation at 37C, the absorbance of the wells was measured at 450 nm. Confocal microscopy H460 and H441 cells were fixed with 3.7% paraformaldehyde and then permeabilized with 0.1% ( w / v ) saponin for 15 min. Cells were co-incubated with primary antibodies against phospho β-catenin and total beta catenin for 12 h at 4 °C, followed by incubating with appropriate Alexa-Fluor-conjugated secondary antibodies for 30 min at 37 °C. Cells were washed and mounted onto glass slides using Vectashield mounting medium containing DAPI. Samples were analysed using a Nikon A1 laser-scanning confocal microscope equipped with a Plan-Apo × 63/1.4 numerical aperture oil lens objective. Acquired images were then analysed using ImageJ software (version 1.41o). KRAS genotyping Genomic DNA from resected lung cancer tissue samples was prepared using a Qiagen Blood and Tissue Kit (Qiagen) according to the manufacturer’s instructions. KRAS mutations were determined using standard RT–PCR and Sanger sequencing protocols for KRAS exon 1, which harbours codons 12 and 13, and exon 2, which harbours codon 61. RT–PCR was performed with 5 ng genomic DNA with 38 cycles of PCR according to the following conditions: 94 °C for 30 s, 56 °C for 30 s and 68 °C for 45 s. PCR products were subsequently purified using ExoSAP-IT PCR purification product (USB/Affymetrix) according to the manufacturer’s instructions. PCR products were then unidirectionally sequenced using the M13 forward primer at the University of Michigan Sequencing Core. Sequence data was analysed for the presence of canonical activating KRAS mutations at codons 12, 13 and 61. Primers used for the PCR reactions are listed in the Supplementary methods . Immunohistochemistry IHC analyses on paraffin-embedded formalin-fixed (FFPE) tumour tissue sections were carried out using the automated DiscoveryXT staining platform from Ventana Medical Systems. All FFPE sections were represented in triplicate on the tissue microarray. The primary rabbit monoclonal LCK antibody was obtained from Cell Signaling (#2,984). Antigen recovery was conducted using heat retrieval and CC1 standard, a high-pH Tris/borate/EDTA buffer (VMSI, catalogue no. 950-124). Slides were incubated with 1:50 of the LCK antibody (Cell Signaling) overnight at room temperature. Primary antibody was detected using the ChromoMap DAB detection kit (VMSI, catalogue no. 760-159) and UltraMap anti-Rb HRP (VMSI, catalogue no. 760-4,315). The anti-Rb HRP secondary antibody was applied for 30 min at room temperature. Slides were counterstained with Hematoxylin for 10 min followed by Bluing Reagent for 5 min at 37 °C. Staining was scored (D.G.B.) as negative (score=0), minimal (score=1), weak (score=2), moderate (score=3) or high (score=4). Accession codes: The mass spectrometry proteomics and phosphoproteomics data have been deposited in the ProteomeXchange Consortium under accession code PXD000439. How to cite this article: Balbin, O. A. et al . Reconstructing targetable pathways in lung cancer by integrating diverse omics data. Nat. Commun. 4:2617 doi: 10.1038/ncomms3617 (2013).